Determination of tyrosinase substrate-binding modes reveals mechanistic differences between type-3 copper proteins Tyrosinase is responsible for the two initial enzymatic steps in the conversion of tyrosine to melanin. Many tyrosinase mutations are the leading cause of albinism in humans, and it is a prominent biotechnology and pharmaceutical industry target. Here we present crystal structures that show that both monophenol hydroxylation and diphenol oxidation occur at the same site. It is suggested that concurrent presence of a phenylalanine above the active site and a restricting thioether bond on the histidine coordinating CuA prevent hydroxylation of monophenols by catechol oxidases. Furthermore, a conserved water molecule activated by E195 and N205 is proposed to mediate deprotonation of the monophenol at the active site. Overall, the structures reveal precise steps in the enzymatic catalytic cycle as well as differences between tyrosinases and other type-3 copper enzymes. Tyrosinase is a di-copper oxidase responsible for the production of melanin in many organisms. It is involved in wound healing, UV protection, detoxification of phenols and more [1] . Mutations in tyrosinase cause albinism in mammals and are associated with melanoma [2] . The active site of all type-3 copper proteins comprises six histidine residues that coordinate the two copper ions CuA and CuB. It is identical among tyrosinases, catechol oxidases (COx) and haemocyanins, yet each member of the family has different function(s). Tyrosinase performs two successive reactions in the presence of molecular oxygen; the hydroxylation of monophenols to form ortho -diphenols (monophenolase activity) and the oxidation of o -diphenols to o -quinones (diphenolase activity). COx are strict diphenolases while haemocyanins bind oxygen and normally do not exhibit catalytic activity, however, some activity was observed in the presence of SDS [3] . The catalytic mechanism of type-3 copper proteins has been studied extensively for the past two decades, recently assisted by the availability of three-dimensional structures [4] , [5] , [6] , [7] , [8] . Based on these structures, it is evident that the differences in function are due to variations in the residues surrounding the substrate-binding pocket. A number of mechanistic studies have also contributed to the current understanding of active site states, substrate inhibition and copper involvement [9] , [10] . However, to date, both mechanistic and structural studies have not provided direct evidence of the catalytic cycle, as visualization of substrates in the active site has not been obtained. Thus, the subtle mechanistic differences between members of this protein family are still undetermined [10] . In this study, we present structural evidence for the identical binding mode of substrates in the active site, as opposed to previous assumptions. This led us to the identification of a more likely mechanism of catalysis, and to an explanation for the difference between tyrosinase and COx. Structures with substrates elucidate reaction mechanism We have determined the crystal structure of tyrosinase from Bacillus megaterium (TyrBm) with substrates bound to the active site. This enzyme’s activity in crystal [7] hampered initial attempts, and the resulting electron density maps lacked evidence of bound molecules. We previously showed that replacing the Cu 2+ with Zn 2+ ions can be performed in TyrBm without structural consequences [7] , while the presence of Zn 2+ ions inhibited the activity of tyrosinase on both monophenols and diphenols [7] , [11] . Based on these observations, we soaked the crystals in ZnCl 2 before soaking them in the substrate solution in order to trap the substrates within the active site of TyrBm in the crystal. This approach was successful, and for the first time high-resolution structures with clear electron density for L -tyrosine or L -Dopa (3,4-dihydroxyphenylalanine) in the active site of tyrosinase were obtained at 2.2 Å resolution ( Fig. 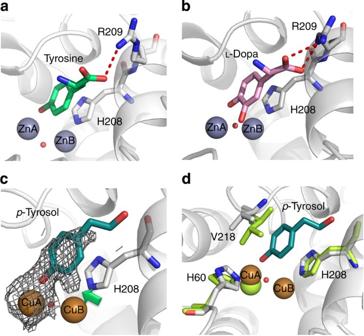Figure 1: Tyrosine,L-Dopa andp-tyrosol at the active site of TyrBm. (a) Tyrosine (green) is observed in the active site. Its carboxyl side chain forms hydrogen bonds with R209. Zinc ions are presented as grey spheres. (b)L-Dopa (pink) is observed in the active site in the same position as tyrosine. (c)p-Tyrosol (teal) with its 2Fo-Fc electron density map (grey wire) contoured at 1.3σ. Copper ions are shown as brown spheres and a water molecule as a red sphere. A green arrow points at the electron density that we propose shows hydroxylation has occurred in crystal. (d) Superposition with the apo-TyrBm structure (light green, PDB code 3NQ0) shows CuA and residues V218 and H60 that have moved, whereas H208 has not. 1 and Table 1 ). Figure 1: Tyrosine, L -Dopa and p -tyrosol at the active site of TyrBm. ( a ) Tyrosine (green) is observed in the active site. Its carboxyl side chain forms hydrogen bonds with R209. Zinc ions are presented as grey spheres. ( b ) L -Dopa (pink) is observed in the active site in the same position as tyrosine. ( c ) p -Tyrosol (teal) with its 2Fo-Fc electron density map (grey wire) contoured at 1.3 σ . Copper ions are shown as brown spheres and a water molecule as a red sphere. A green arrow points at the electron density that we propose shows hydroxylation has occurred in crystal. ( d ) Superposition with the apo-TyrBm structure (light green, PDB code 3NQ0) shows CuA and residues V218 and H60 that have moved, whereas H208 has not. Full size image Table 1 Data collection and refinement statistics. Full size table The TyrBm structure with bound L -tyrosine (TyrBm:T) is presumed to be in the enzymes’ met form [1] , [7] , [10] . As expected [12] , [13] , the tyrosine hydroxyl group is directed towards ZnA (at the equivalent position of CuA) at a distance of 1.9 Å and its benzyl ring is oriented through hydrophobic π–π interactions with H208 ( Fig. 1a ). In this orientation, the ortho position is electrophilic and directed towards the proposed oxygen species binding site located between CuA and CuB. Previous studies have suggested that diphenols are oriented towards CuB [9] , [10] , thus relating each of the two activities to a different Cu ion. This suggestion is also based on the structure of COx in which CuA is shielded by a bulky phenylalanine residue (F261) and only the diphenolase activity is observed. Previous results from our laboratory, using directed evolution on TyrBm, showed that when access to CuB is hindered by mutation R209H, the diphenolase activity decreases while the monophenolase activity increases [14] . However, the crystal structure at 2.2 Å resolution of TyrBm with L -Dopa in the active site (TyrBm:D; Table 1 ) unequivocally shows that the diphenol binds to ZnA in the same orientation as tyrosine, assisted by interactions with H208 ( Fig. 1b and Supplementary Fig. 1 ). This result indicates that both the hydroxylation and oxidation activities occur without significant binding site reorganization. The question that arises, therefore, is what differentiates the activity of tyrosinases and the homologous COx? Superposition of TyrBm:T and TyrBm:D, with sweet potato COx [4] (PDB code 1BUG), indicates that both tyrosine and L -Dopa can be positioned in the active site, considering the location of F261 of COx ( Fig. 2 ). However, the flexibility of F261 is restricted owing to the thioether bond fixing one of the histidines [4] (which is flexible in bacterial tyrosinases [6] , [15] ), and therefore it cannot allow for any substrate rotation during the reaction. During the monophenolase reaction, a rotation of the tyrosine is suggested to occur, allowing the electrophilic attack that leads to hydroxylation [12] , [16] ( Fig. 3 ). This was suggested by Decker and colleagues [16] , and was further confirmed by using molecular dynamics by Deeth and Dietrich [13] . These studies, however, have not dealt with the molecular mechanism of reaction in the case where the diphenol enters the active site. We suggest that since the reaction on L -Dopa does not involve an electrophilic attack but only the oxidation of the two hydroxyl groups, the rotation in this case is not necessary and does not occur. Thus, the diphenolase reaction in COx can be performed despite the partial blocking of the active site by the perturbing phenylalanine. 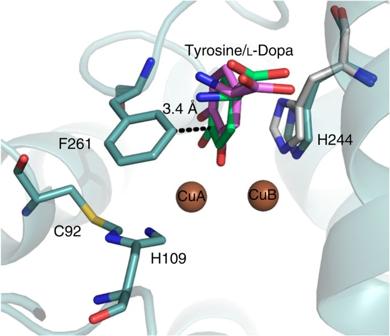Figure 2: Superposition of TyrBm substrates in the active site of COx (PDB code 1BUG; ref.4). Tyrosine (in green) and L-Dopa (in pink) can be positioned in the active site of COx considering the distance shown from F261 (in teal). H244, of COx (in teal), is positioned similarly to H208 of TyrBm (in grey). H109 of COx is restricted by the thioether bond with C92. Figure 2: Superposition of TyrBm substrates in the active site of COx (PDB code 1BUG; ref. 4 ). Tyrosine (in green) and L-Dopa (in pink) can be positioned in the active site of COx considering the distance shown from F261 (in teal). H244, of COx (in teal), is positioned similarly to H208 of TyrBm (in grey). H109 of COx is restricted by the thioether bond with C92. 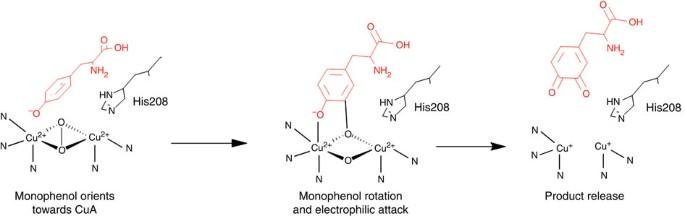Figure 3: Structure-supported monophenol hydroxylation mechanism based on Deeth and Dietrich13. During the monophenolase reaction, a rotation of tyrosine is suggested to occur, allowing the electrophilic attack that leads to hydroxylation. Full size image Figure 3: Structure-supported monophenol hydroxylation mechanism based on Deeth and Dietrich [13] . During the monophenolase reaction, a rotation of tyrosine is suggested to occur, allowing the electrophilic attack that leads to hydroxylation. Full size image Substrate deprotonation scenario The newly obtained TyrBm:T and TyrBm:D structures reveal an additional important element of the reaction mechanism. It has been suggested that substrates bind to the active site as a phenolate, therefore a mechanism of deprotonation [16] by the enzyme is expected. This proton needs to then be returned to the active site for the generation of water and the release of the quinone product. A number of options have been previously suggested for the identity of the deprotonating base [6] , [16] . The highly conserved E195 has been suggested as the potential base; however, its distance from the active site (7 Å) is too great for such activity. Examination of the vicinity of this residue in TyrBm:T and TyrBm:D (as well as over 30 other TyrBm structures we have determined) showed that almost invariably, a water molecule is located bound equidistant between the E195 carboxyl group and the conserved N205 carbonyl group ( Fig. 4 ) previously shown to be vital for activity and copper uptake [17] . A similar water molecule is also observed in the structures of sweet potato COx (1BT3; ref. 4 ), Streptomyces tyrosinase (1WX2; ref. 6 ), Agaricus bisporus tyrosinase (2Y9W; ref. 8 ) and Manduca sexta tyrosinase (3HHS; ref. 5 ). We propose that this conserved water molecule is activated by E195 and N205, and serves as the deprotonating base. The involvement of water molecules or hydroxide ions in enzyme catalysis has been previously shown in several studies with other enzymes [18] , [19] , [20] . A recent QM calculation study performed by Siegbahn and Borowski [21] examined the reaction mechanism and suggested a similar deprotonation scenario. They showed that it is energetically feasible to move the proton from tyrosine through the water molecule to the glutamate residue (E195). They also considered the involvement of three additional residues in this scenario that are also highly conserved, R191, N192 and D178, and which stabilize the water molecule through E195 ( Fig. 4 ). Attempts to mutate E195 to arginine or leucine resulted in insoluble protein further strengthening the importance of this conserved residue. 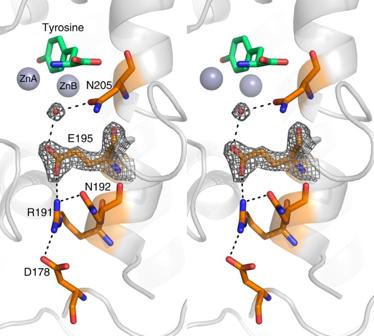Figure 4: Structure-supported deprotonation scenario. Stereoview of structure TyrBm:T in which a conserved water molecule is shown oriented by E195 and N205 (orange) with their 2Fo-Fc electron density map (grey wire) contoured at 2.2σ. Conserved residues R191 N192 and D178 (orange) are also assumed to be involved in the deprotonation scenario. All dashed lines represent a distance of ~3.0 Å. Figure 4: Structure-supported deprotonation scenario. Stereoview of structure TyrBm:T in which a conserved water molecule is shown oriented by E195 and N205 (orange) with their 2Fo-Fc electron density map (grey wire) contoured at 2.2 σ . Conserved residues R191 N192 and D178 (orange) are also assumed to be involved in the deprotonation scenario. All dashed lines represent a distance of ~3.0 Å. Full size image TyrBm active structure presents product formation In order to obtain a substrate in the active site in the presence of Cu 2+ , we soaked crystals with p -tyrosol, which TyrBm hydroxylates relatively slowly in comparison with tyrosine. The TyrBm p -tyrosol structure (TyrBm:P) with Cu 2+ in the active site was determined at a resolution of 2.5 Å ( Fig. 1c and Table 1 ). Tyrosol is observed in both subunits in the asymmetric unit, directed towards CuA and oriented by His208, as was the case for tyrosine. In one of the subunits, clear electron density at the ortho position of the p -tyrosol is observed ( Fig. 1c ), which we interpret as a snapshot of hydroxytyrosol (the diphenol), or perhaps even the final quinone product. Two major differences in the active site are seen in the TyrBm:P structure: (i) V218, the residue in the loop above the active site, moves 1.4 Å to allow substrate entrance, confirming its role as recently suggested [15] ; and (ii) CuA moves 1.0 Å towards the hydroxyl of the bound substrate ( Fig. 1d ). Our results support findings by Kleifeld et al. [22] that showed that during different steps along catalytic cycles, metal ions may accommodate alternative locations. We present here for the first time a detailed structure-based mechanism of tyrosinase. The structures of TyrBm with bound substrates presented here confirm that monophenols and diphenols bind identically at the active site towards CuA. Based on these structures and on a number of recent studies [13] , [15] , [16] , we suggest that although both mono- and diphenols orient within the active site in the same way, only monophenols rotate during the reaction. This fact enables to differentiate between enzymes with both mono- and diphenolase activities and those that are strict diphenolases. Thus, in sweet potato COx and similar enzymes, two constraints need to coexist in order to prevent monophenolase activity: (i) a bulky residue above the active site (such as F261) and (ii) a restricting thioether bond on the active site histidine coordinating CuA. The presence of both constraints prevents substrate axial to equatorial rearrangement needed for monophenolase hydroxylation, but allows for the oxidation of a diphenol. Consequently, TyrBm variant V218F can hydroxylate tyrosine owing to the absence of a thioether bond [15] , and tyrosinase from A. bisporus performs hydroxylation despite the thioether bond because of the presence of V283 above the active site [8] . This provides a compelling and structurally founded explanation for the long-lasting debate on the different activities of type-3 copper proteins. Another major issue discussed in the literature concerning the catalytic cycle of tyrosinases has been the deprotonation of the entering substrates [16] , which is in fact the initial step of the reaction. We suggest here that the base that deprotonates the substrate is a conserved hydroxide or water molecule oriented and activated by two highly conserved residues, a glutamic acid and an asparagine. Importantly, substrate deprotonation has been suggested to be involved in diphenol substrate inhibition or suicide inactivation [9] , [23] . The suicide inactivation pathway of diphenols is apparently facilitated by the incorrect proton transfer to the active site peroxide instead of to an adjacent base. In light of the new evidence showing that both substrates bind to CuA, the existence of such an inactivation mechanism also explains the ability to influence the monophenolase/diphenolase activity ratio, as in TyrBm mutants [14] , [15] , [17] . Finally, the formation of product within the TyrBm structure has been presented. The use of p -tyrosol as a substrate, which is hydroxylated at a slower rate than tyrosine, enabled us not only to determine the crystal structure of the TyrBm:substrate complex in the presence of Cu 2+ in the active site, but also to observe product formation in the crystal. The fact that tyrosine in the TyrBm:T structure is observed in a very similar orientation as p -tyrosol in the TyrBm:P structure, supports our claim that Zn 2+ in the active site may only prevent protein activity but not substrate binding. Purification and crystallization of tyrosinase from TyrBm A tyrosinase producing TyrBm was isolated from soil samples and the gene encoding for the tyrosinase was cloned into Escherichia coli BL21. The enzyme was expressed, purified and crystalized as previously described [7] , [24] , [25] . Briefly, E. coli cells were grown overnight at 37 °C in 0.5 l of TB medium (tryptone 1.2%, yeast extract 2.4%, glycerol 0.4% (w/v) and potassium phosphate buffer 89 mM) and then harvested by centrifugation (8,000 g for 10 min at room temperature). Cells were treated twice in a pressure cell (French Press, Spectronic Instruments Inc., Rochester, NY, USA) and cell debris was removed by centrifugation (16,000 g for 20 min at 15 °C). The supernatant containing TyrBm was applied to a Ni(II)-bound affinity column and eluted with an appropriate buffer (20 mM Tris–HCl, pH 7.5, 500 mM NaCl and 500 mM imidazole). Crystallization was performed using the hanging-drop vapour diffusion method at 293 K. Drops consisting of 2 μl protein solution (2 mg ml −1 ) and 2 μl of the mother liquor were equilibrated against a 600-μl reservoir containing 18% PEG 8000 and 0.1 M cacodylic acid, pH 6.5. Substrate binding in crystal In order to trap ligands in the active site, mature crystals were soaked overnight in 1 mM of either CuSO 4 or ZnCl 2 and subsequently in 1 mM of the appropriate ligand ( L -tyrosine, p -tyrosol and L -Dopa). To ensure maximal occupancy, an additional soaking of the ligand for 1–5 min was performed before crystal freezing. Data collection and structure determination X-ray diffraction data was collected at the European Synchrotron Radiation Facility, Grenoble, France, at beamlines ID14-1 and ID 23-1. All data were indexed, integrated, scaled and merged using Mosflm and Scala [26] . The initial structure of TyrBm was solved by molecular replacement using Phaser [27] and the coordinates of earlier determined TyrBm structure (PDB code 3NM8). A single solution was obtained for two monomers in the asymmetric unit. Refinement was performed using Phenix [28] coupled with rounds of manual model building, real-space refinement and structure validation performed using COOT [29] . Data collection, phasing and refinement statistics are presented in Table 1 . Accession codes: Coordinates and structure factors of TyrBm have been deposited in the RCSB Protein Data Bank under accession code 4P6R for TyrBm:T, 4P6S for TyrBm:D and 4P6T for TyrBm:P. How to cite this article: Goldfeder, M. et al. Determination of tyrosinase substrate-binding modes reveals mechanistic differences between type-3 copper proteins. Nat. Commun. 5:4505 doi: 10.1038/ncomms5505 (2014).